Photoredox-catalyzed branch-selective pyridylation of alkenes for the expedient synthesis of Triprolidine Alkenylpyridines are important pharmaceutical cores as well as versatile building blocks in organic synthesis. Heck reaction represents one of the most powerful platform for the construction of aryl-substituted alkenes, nevertheless, examples for Heck type coupling of alkenes with pyridines, particularly with branched selectivity, remain elusive. Here we report a catalytic, branch-selective pyridylation of alkenes via a sulfinate assisted photoredox catalysis. This reaction proceeds through a sequential radical addition/coupling/elimination, by utilizing readily available sodium sulfinates as reusable radical precursors as well as traceless elimination groups. This versatile protocol allows for the installation of important vinylpyridines with complete branched selectivity under mild conditions. Furthermore, this catalytic manifold is successfully applied to the expedient synthesis of Triprolidine. Pyridine is recognized as one of the most important heterocycles in pharmaceuticals, agrochemicals, and bioactive natural products [1] , [2] . Alkenylpyridines, an important subunit of pyridines, also serve as versatile synthetic building blocks for complex pyridines [3] , [4] , as well as important ligand scaffolds in the area of catalysis (Fig. 1a ) [5] . As a result, the efficient and selective assembly of alkenylpyridines from readily available starting materials has drawn intensive attentions of chemists [6] , [7] , [8] , [9] , [10] . Fig. 1 Design of catalytic and branch-selective alkene–pyridine coupling via photoredox catalysis. a Importance of alkenylpyridines. b Photocatalyzed alkylations of pyridines. c Design of branch-selective alkenylation of pyridines via photoredox catalysis Full size image Alkenes are one of the most ubiquitous material in organic synthesis. The cross-coupling of alkenes and aryl halides in the presence of palladium catalyst, the Heck reaction [11] , [12] , [13] , is a powerful protocol for the construction of aryl-substituted alkenes. Nevertheless, there are few examples of Heck coupling of alkenes with pyridines, probably due to the potential coordination between the nitrogen atom and metal catalyst [14] , [15] , [16] , [17] , [18] , [19] . Alternatively, several examples of Pd-catalyzed cross-coupling of alkenes with pyridine N -oxides have been reported, while only delivering vinylpyridine derivatives with linear selectivity [20] , [21] , [22] , [23] . To the best of our knowledge, catalytic alkene–pyridine couplings with branch selectivity, the control of which remains a big challenge in Heck couplings [24] , [25] , [26] , is unknown. Recently, radical-based chemistry provides an alternative platform to address this challenge. Particularly, the groups of MacMillan, Jui, and others [27] , [28] , [29] , [30] , [31] , [32] , [33] , [34] , [35] , [36] , [37] , [38] , [39] , [40] , [41] , [42] , [43] , [44] , [45] , [46] have successfully demonstrated that visible light photocatalyzed cross-couplings of pyridines to access to alkylated pyridines under mild conditions, by taking advantage of unique reactivity of open-shell pyridyl radical species (Fig. 1b ). While significant advances, no examples of vinylation of pyridines via pyridyl radical species has been reported. Herein, we demonstrate an alternative protocol, through a sequential radical addition/radical coupling/elimination pathway, to access vinylpyridines from readily available alkenes with complete branch selectivity (Fig. 1c ). This reaction takes advantage of a synergistic combination of visible light-induced photoredox catalysis and a catalytic radical precursor, providing an effective and selective strategy for the synthesis of α-vinylpyridines under mild conditions. Design plan We hypothesized that sodium sulfinates would be the ideal reusable radical precursors, due to the unique properties of which: (i) sufinates have been recently employed as efficient sulfonyl coupling partners in photoredox catalysis [47] , [48] , [49] , [50] , [51] , [52] , [53] , [54] , [55] , [56] , [57] , [58] , [59] , [60] , [61] , [62] ; (ii) it is well known that the alkyl sulfones would be prone to undergo desulfonylation under basic conditions [63] , [64] , [65] . As depicted in Fig. 2 , we envisioned that a single-electron reduction between photoexcited *Ir(ppy) 3 2 { E 1/2 red [*Ir III /Ir IV ] = –1.73 V vs. SCE } [66] and cyanopyridine 3 ( E 1/2 red = –1.75 V vs. SCE in CH 3 CN) [67] could be feasible under specific conditions, generating pyridyl radical anion species 3 and the oxidizing Ir IV 5 . We hypothesized that Ir IV 5 { E 1/2 red [Ir IV /Ir III ] = +0.77 V vs. SCE} [66] , [68] could affect the oxidation of sodium methanesulfinate 6 ( E 1/2 red = +0.50 V vs. SCE) (see Supplementary Fig. 2 ) to form sulfonyl radical 7 and regenerate the ground-state Ir III catalyst 1 . The electrophilic sulfonyl radical 7 would subsequently undergo facile radical addition to alkene to generate the nucleophilic benzylic radical 9 . At this stage, we envisioned that radical–radical coupling between the transient benzylic radical 9 and the persistent pyridyl radical anion 4 would forge β-sulfonyl pyridine 10 [32] , [33] , [34] , [35] , [36] , [37] , [38] , [39] , [40] , [41] , [42] , [43] , [44] , [45] , [46] . Due to the acidity of the benzylic proton and the good leaving ability of sulfone, alkyl sulfone 10 would be expected to undergo E1 elimination with the assistant of base, furnishing the final branched alkenylpyridine product 11 , as well as sulfinate 6 that could be recycled. Fig. 2 Proposed mechanism. 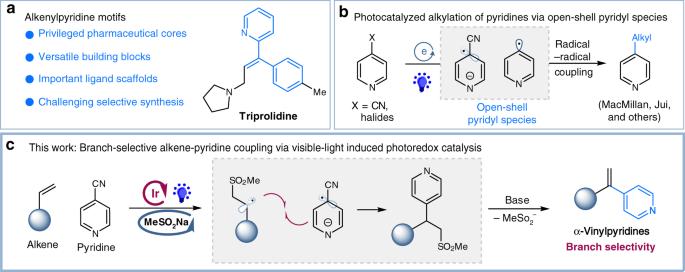Fig. 1 Design of catalytic and branch-selective alkene–pyridine coupling via photoredox catalysis.aImportance of alkenylpyridines.bPhotocatalyzed alkylations of pyridines.cDesign of branch-selective alkenylation of pyridines via photoredox catalysis Possible reaction pathway utilizing sulfinate as a promoter Full size image Optimization study Our investigation into this photoredox cascade protocol began with exposure of 1-( tert -butyl)-4-vinylbenzene 12 and 4-cyanopyridine 3 to a 90 W blue light-emitting diode (LED) in the presence of catalytic amounts of Ir(ppy) 3 (5 mol%) and readily available MeSO 2 Na (30 mol%) (Table 1 ). In the presence of a stoichiometric amount of 1,8-diazabicyclo[5.4.0]undec-7-ene (DBU) as base; pleasingly, we found that the branched vinylpyridine product could be obtained in 69% yield (entry 1). The nature of sodium sulfinates was found to have an important effect to the reaction efficiency. Generally, electron-poor aryl sulfinates, which are better leaving groups, afforded higher efficiency than electron-rich ones (entries 2–6). And, comparable yields were obtained when para -chlorophenyl sulfinate was employed as the co-catalyst (entry 4). Gratifyingly, increasing the photocatalyst loading to 5 mol% provided the optimal yield of product (entry 7). Control experiments indicated that photocatalyst, sulfinate, and light were all essential to this transformation, as no desired products were observed in the absence of either photocatalyst, sulfinate, or light (entries 8–10). While conducting the reaction in the absence of DBU afforded the expected product in 18% yield, probably due to the basic condition in the presence of MeSO 2 Na (entry 11). Interestingly, a trace amount of C2-substituted product 13′ , which is assumed to be formed by the S N Ar reaction of cyanopyridine with alkyl radical, was observed under the reaction conditions [69] . Table 1 Optimization of reaction conditions a Full size table Substrate scope With the optimal conditions in hand, we next explored the generality of this transformation with respect to alkene component using 4-cyanopyridine as the coupling partner. As shown in Fig. 3 , styrenes incorporating electron-donating and electron-withdrawing substituents readily underwent the desired radical addition/coupling/elimination cascade reactions, furnishing branched vinylpyridines in good to high yields (products 13 – 32 , 53–86% yields). The mild conditions tolerate a wide range of functional groups, including ethers, amides, esters, nitriles, chlorides, bromides, ketones, and amines (products 16 – 20 , 22 – 31 , 53–73% yields). Moreover, ortho substituents (Me, F, Cl) on the aryl ring were compatible in this manifold, albeit with slightly diminished yields (products 30 – 32 , 53–68% yields). Furthermore, this catalytic protocol was applicable to other aryl and heteroaryl alkenes, in the form of naphthalene, benzofuran, thiophene, and thiazole, furnishing the corresponding products in moderate yields (products 33 – 36 , 56–78% yields). It should be noted that both cyclic (e.g., 1,2-dihydronaphthalene) and acyclic (e.g., trans -β-methylstyrenes and benzyl ether of cinnamyl alcohol) internal alkenes were found to be viable substrates, delivering the corresponding alkenylpyridines with exclusive selectivity at the benzylic positions, respectively (products 37 – 40 , 69–75% yields). Finally, styrenes derived from drugs or natural products, including oxaprozin, nonivamide, hymecromone, estrone, and indomethacin, could be successfully employed to furnish the desired products in moderate to good yields (products 41 – 45 , 48–89% yields), further highlighting the potential synthetic utility of this new protocol. Notably, piperine, a naturally occurring alkaloid, underwent selective pyridylation with synthetic useful yields (product 46 , 49% yield). Nevertheless, un-activated alkenes were ineffective under the reaction conditions, and most of alkene materials remained, probably due to their weaker electrophilic nature. Fig. 3 Substrate scope of olefins. Reaction conditions: Ir(ppy) 3 (5 mol%), MeSO 2 Na (30 mol%), alkene (0. mmol), 4-cyanopyridine (2.0 equiv. ), DBU (3 equiv. ), MeCN/EtOH (1:1), 90 W blue light-emitting diode (LED), 40 °C, 24 h. All cited yields are isolated yields. a Employed with 4-Cl-C 6 H 4 SO 2 Na (1.0 equiv). b Employed with 4-Cl-C 6 H 4 SO 2 Na (0.5 equiv.). c The ratio was determined by proton nuclear magnetic resonance ( 1 H NMR) analysis Full size image We next sought to explore the scope regarding cyanopyridines (Fig. 4 ). Nevertheless, we found that only 4-cyanopyridines with alkyl and/or aryl substituents at the 2-positions underwent the desired couplings with moderate efficiency under the standard conditions (products 47 – 48 , and 50 , with yields around 50%). Pleasingly, employing a stoichiometric amount of 4-chlorophenyl sulfinate as the radical precursor and NH 4 Cl as the additive could improve the reaction efficiency. 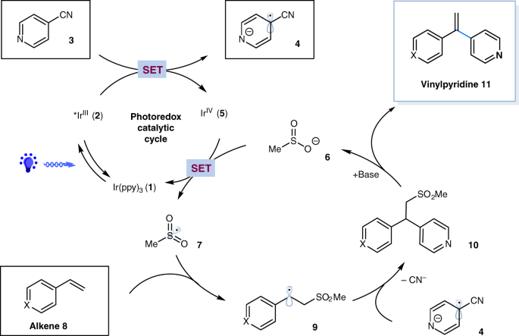Fig. 2 Proposed mechanism. Possible reaction pathway utilizing sulfinate as a promoter Under the modified conditions, a wide range of cyanopyridines could be successfully employed, furnishing the desired α-vinylpyridines in moderate to good yields (products 47 – 58 , 71–86% yields). Notably, halogen atoms remained intact under the photocatalytic conditions, offering useful handles for further synthetic manipulations (products 53 – 56 , 71–72% yields). Interestingly, 3,4-dicyanopyridine underwent selective coupling at C4 (product 58 , 86% yield), while 2,4-dicyanopyridine afforded a mixture of regioisomeric products (product 51 , 81% yield, r.r. = 1.7:1). Ortho substituents on the pyridines have no deleterious effect to the coupling/elimination efficiency (products 56 – 58 , 71–86% yields). Moreover, unprotected azaindole nitrile also was a viable substrate (product 58 , 73% yield). Notably, 1-cyanoisoquinoline and 2-cyanopyridines also underwent the selective alkenylation smoothly, delivering the corresponding vinylquinoline and vinylpyridines with moderate efficiency (products 13′ , 60 – 63 , 69–85% yields). Pleasingly, performing the photocatalytic reaction on a 5 mmol scale afforded product 63 with comparable efficiency (see Supplementary Fig. 1 for details). Fig. 4 Substrate scope of pyridines. Reaction conditions: Ir(ppy) 3 (1 mol%), 4-Cl-PhSO 2 Na (1.0 equiv. ), styrene (0.2 mmol), cyanopyridine (2.0 equiv. ), NH 4 Cl (2 equiv. ), base (6 equiv. ), MeCN/EtOH, 90 W blue light-emitting diode (LED, 40 °C, 2 h. All cited yields are isolated yields. a The ratio was determined by 1 H NMR analysis. b Reaction performed on a 5 mmol scale. see Supplementary Fig. 1 for details. Ar = 4- tert -butylphenyl Full size image To demonstrate the synthetic application of this sequential photoredox protocol, we have accomplished the expedient synthesis of Triprolidine, a top-selling antihistamine that used for allergies [70] , [71] . As shown in Fig. 5a , Pd-catalyzed amination of commercially available allylic 4-methylcinnamic alcohol 64 gave the allylic amine precursor 65 in 86% yield [72] . Reaction of 65 with simple 2-cyanopyridine under our photocatalytic conditions directly delivered Triprolidine in a simple and one-pot operation with a synthetic useful yield (48% yield). Notably, a 5 mmol scale synthesis of Triprolidine was performed, albeit with slightly decreased efficiency (35% yield). Furthermore, subjection of allylic amine 65 to the photocatalytic condition, yielding the desired pyridyl product 66 , a precursor for drug pheniramine [73] through one-step hydrogenation [74] , with 42% yield (Fig. 5b ). 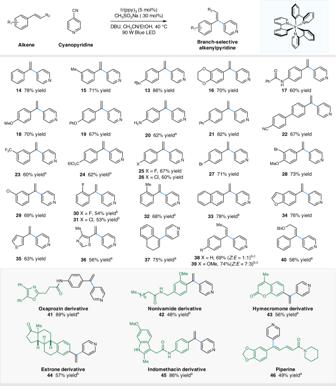Fig. 3 Substrate scope of olefins. Reaction conditions: Ir(ppy)3(5 mol%), MeSO2Na (30 mol%), alkene (0. mmol), 4-cyanopyridine (2.0 equiv.), DBU (3 equiv.), MeCN/EtOH (1:1), 90 W blue light-emitting diode (LED), 40 °C, 24 h. All cited yields are isolated yields.aEmployed with 4-Cl-C6H4SO2Na (1.0 equiv).bEmployed with 4-Cl-C6H4SO2Na (0.5 equiv.).cThe ratio was determined by proton nuclear magnetic resonance (1H NMR) analysis Fig. 5 Synthesis of Triprolidine. a One-pot synthesis of Triprolidine via photoredox catalysis. b Synthesis of pheniramine precursor Full size image Mechanistic studies To further probe the mechanism proposal of this photocatalytic reaction, we performed Stern–Volmer fluorescence quenching studies. As shown in Supplementary Fig. 3 , only cyanopyridine was found to quench the excited state of *Ir(ppy) 3 , while no significant quenching was observed in the presence of sulfinate or DBU, lending support for our proposed oxidative quenching pathway (Fig. 2 ). Next, investigation of the intermediacy of a sulfonyl radical was conducted (Fig. 6 ). Reaction of vinylcyclopropane 68 with MeSO 2 Na and 4-cyanopyridine in the presence of Ir(ppy) 3 and DBU afforded product 69 , which could be formed through a sequential sulfonyl addition/ring opening/radical coupling protocol (Fig. 6a ). Furthermore, the reaction of styrene and 4-chlorophenyl sulfinate, in the absence of DBU, gave 24% of the desired vinylpyridine product 16 as well as 65% of isolable β-sulfonyl pyridine 70 . As expected, treatment of 70 with DBU gave vinylpyridine 16 in 94% yield (Fig. 6b ). These results further supported the intermediacy of a sulfonyl radical species in the transformation. Regarding the coupling step for forging the C–pyridine bond, nevertheless, we cannot rule out alternative pathway that proceeds via S N Ar reaction of pyridine with alkyl radical 9 , particularly with the observation of a trace amount of C2-substituted product (see Supplementary Fig. 4 for this alternative pathway). Fig. 6 Mechanistic studies. a Radical clock experiment. b Isolation of alkyl sulfone intermediate Full size image In conclusion, we have developed an efficient strategy for branch-selective, formal alkene–pyridines cross-coupling via sulfinate-assisted photoredox catalysis. This versatile protocol utilizes a sequential radical addition, radical coupling, and β-elimination protocol, allowing for the construction of branched alkenylpyridines from simple starting material under mild conditions. Notably, an expedient and an operationally simple, one-pot synthesis of Troprilidine has been successfully achieved through this photocatalytic manifold. General procedure for the branch-selective alkenylpyridylation reaction To a flame-dried 20 mL reaction vial was charged with Ir(ppy) 3 (1.0 mol%), MeSO 2 Na (30 mol%), 4-cyanopyridine (0.4 mmol, 2.0 equiv. 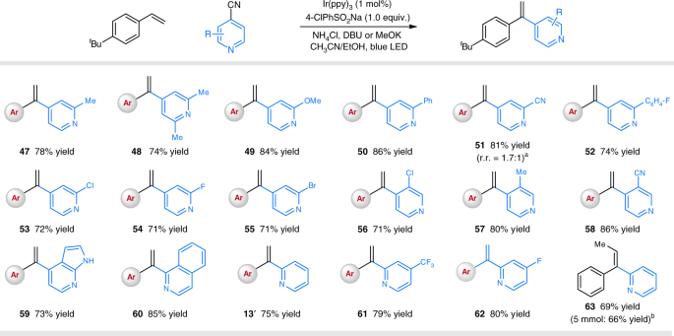Fig. 4 Substrate scope of pyridines. Reaction conditions: Ir(ppy)3(1 mol%), 4-Cl-PhSO2Na (1.0 equiv.), styrene (0.2 mmol), cyanopyridine (2.0 equiv.), NH4Cl (2 equiv.), base (6 equiv.), MeCN/EtOH, 90 W blue light-emitting diode (LED, 40 °C, 2 h. All cited yields are isolated yields.aThe ratio was determined by1H NMR analysis.bReaction performed on a 5 mmol scale. see Supplementary Fig.1for details. Ar = 4-tert-butylphenyl 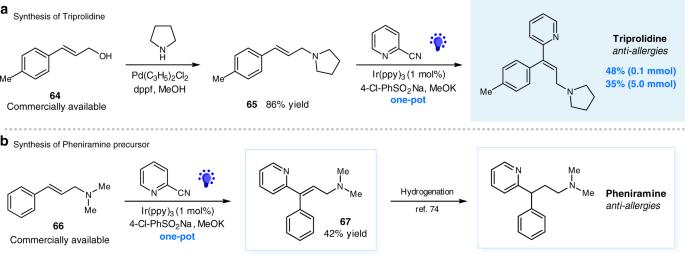Fig. 5 Synthesis of Triprolidine.aOne-pot synthesis of Triprolidine via photoredox catalysis.bSynthesis of pheniramine precursor 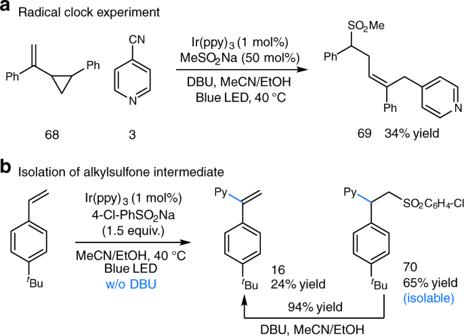Fig. 6 Mechanistic studies.aRadical clock experiment.bIsolation of alkyl sulfone intermediate ), and a magnetic stir bar. MeCN/EtOH (1:1 v/v) [0.02 M] was added, and the vial was capped. The reaction mixture was degassed by nitrogen sparging for 15 min, followed by the addition of alkenes (0.2 mmol, 1.0 equiv.) and DBU (0.6 mmol, 3.0 equiv.). The reaction mixture was then irradiated with a 90 W blue LED for 24 h at 40 °C. The reaction mixture was concentrated in vacuo and then quenched with water, extracted with ethyl acetate. The combined organic layers were dried with MgSO 4 , filtered, and concentrated in vacuo. The crude material was purified by flash chromatography to afford the products. See Supplementary Methods for further experimental details.